Kinase fusions are frequent in Spitz tumours and spitzoid melanomas Spitzoid neoplasms are a group of melanocytic tumours with distinctive histopathological features. They include benign tumours (Spitz naevi), malignant tumours (spitzoid melanomas) and tumours with borderline histopathological features and uncertain clinical outcome (atypical Spitz tumours). Their genetic underpinnings are poorly understood, and alterations in common melanoma-associated oncogenes are typically absent. Here we show that spitzoid neoplasms harbour kinase fusions of ROS1 (17%), NTRK1 (16%), ALK (10%), BRAF (5%) and RET (3%) in a mutually exclusive pattern. The chimeric proteins are constitutively active, stimulate oncogenic signalling pathways, are tumourigenic and are found in the entire biologic spectrum of spitzoid neoplasms, including 55% of Spitz naevi, 56% of atypical Spitz tumours and 39% of spitzoid melanomas. Kinase inhibitors suppress the oncogenic signalling of the fusion proteins in vitro . In summary, kinase fusions account for the majority of oncogenic aberrations in spitzoid neoplasms and may serve as therapeutic targets for metastatic spitzoid melanomas. Melanocytic neoplasms comprise several tumour types that are characterized by distinct clinical, pathological and genetic features. The clinical course of melanocytic tumours may be indolent (benign naevi), aggressive (malignant melanomas) or intermediate (melanocytic tumours of uncertain malignant potential). In 1948, Sophie Spitz [1] coined the term ‘melanoma of childhood’ for a group of melanocytic skin tumours composed of spindled or epithelioid melanocytes that developed predominantly in children and adolescents. It later became clear that these tumours could also arise later in life, and that the majority of these neoplasms behaved in an indolent manner, which led to the introduction of the term ‘Spitz naevus’ to indicate their benign nature. Malignant tumours with spitzoid histological features were termed ‘spitzoid melanomas’, and these tumours often showed aggressive clinical behaviour with widespread metastasis, similar to conventional melanomas. Tumours with histological features overlapping those of Spitz naevi and spitzoid melanoma have been termed ‘atypical Spitz tumours’. Atypical Spitz tumours have the capacity to metastasize, but this is usually limited to the regional lymph nodes, and has little effect on patient survival [2] , [3] . The genomic alterations in the majority of spitzoid neoplasms are not known, and they lack mutations in melanoma-associated oncogenes such as NRAS, KIT, GNAQ or GNA11 (ref. 4 ). However, subsets of spitzoid neoplasms characterized by distinct histopathological features show HRAS mutations [5] , or BRAF mutations combined with bi-allelic BAP1 loss [6] , [7] , suggesting that activation of kinase pathways plays an important role in the pathogenesis of these tumours. Identification of additional genetic events in kinase pathways may contribute to a better understanding of the pathogenesis of spitzoid neoplasms, and may facilitate the development of effective targeted therapies for metastasizing tumours, as illustrated by the success of small molecule kinase inhibitors in prolonging the lives of patients with a broad range of malignancies [8] , [9] , [10] , [11] . For diagnostic reasons, spitzoid neoplasms are usually formalin-fixed and paraffin-embedded (FFPE) in their entirety, and nucleic acids isolated from FFPE tissue are typically degraded and of suboptimal quality. In addition, the percentage of neoplastic cells in spitzoid neoplasms is frequently low due to the presence of varying numbers of admixed non-neoplastic lymphocytes, fibroblasts and keratinocytes. The suboptimal quality of extracted nucleic acids and the low proportion of neoplastic melanocytic cells make the identification of genetic aberrations in spitzoid neoplasms challenging and a high sequencing coverage is necessary. In this study, we therefore used a massively parallel sequencing approach with high sequencing coverage for previously described cancer genes to investigate genetic aberrations in spitzoid neoplasms. Here our genomic analysis of 140 spitzoid neoplasms reveals gene rearrangements of the kinases ROS1 (17%; n =24), NTRK1 (16%; n =23), ALK (10%; n =14), BRAF (5%; n =7) and RET (3%; n =4) resulting in in-frame kinase fusions. These kinase fusions occur across the entire biological spectrum of spitzoid neoplasms, including Spitz naevi (55%, fusions in 41 of 75 cases), atypical Spitz tumours (56%; fusions in 18 of 32 cases) and spitzoid melanomas (39%; fusions in 13 of 33 cases). The chimeric proteins appear in a mutually exclusive pattern, are constitutively active, stimulate oncogenic signalling pathways, are tumourigenic and may serve as diagnostic markers and as therapeutic targets for aggressive or metastasizing Spitz tumours. 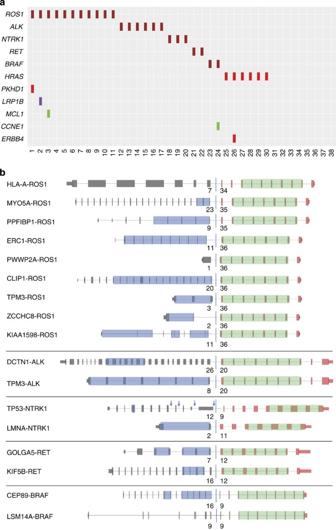Figure 1: Genomic aberrations identified in 38 spitzoid neoplasms by targeted sequencing. (a) The columns denote the samples, the rows denote genes, brown squares represent gene fusions, red squares symbolize point mutations and indels, green squares denote gene amplifications and purple squares indicate truncating mutations. The identified fusion genes andHRASmutations were mutually exclusive in 38 spitzoid neoplasms. Mutations inPKHD1, ERBB4,LRP1B, and amplifications ofMCL1andCCNE1are of unknown significance and co-occurred with kinase fusions and HRAS mutations. (b) Illustration of the distinct fusion genes for theROS1,ALK,NTRK1,RETandBRAFrearrangements. The grey bars represent the exons of the genes, the numbers below the bars the exon number and the blue line the predicted breakpoints. The green shaded areas indicate the kinase domain and the blue shaded areas the coiled-coil domain of the fusion gene product. In theTP53–NTRK1fusion transcript, multiple breakpoints spanning exon 8–12 ofTP53were predicted. Identification of kinase fusions We investigated genomic alterations in a discovery cohort of 30 Spitz naevi and 8 atypical Spitz tumours by targeted massively parallel sequencing ( Supplementary Table 1 summarize the clinical, histopathological and genetic data). For targeted DNA sequencing, we sequenced 3,230 exons from 182 cancer-related genes and 37 introns of 14 genes commonly rearranged genes in cancer. We obtained an average unique coverage of 997 × , with 99.96% of exons being sequenced at ≥100 × coverage. In addition, we performed targeted transcriptome sequencing for 612 transcripts of kinases and kinase-related genes and achieved an average of 56,588,548 unique read pairs per spitzoid neoplasm. Six tumours (16%) harboured HRAS c.182A>T (p.Q61L) mutations and exhibited histopathologic features characteristic of the previously described HRAS -mutant Spitz naevus variant [5] . Additionally, we found mutations in PKHD1, ERBB4 , LRP1B and amplifications of MCL1 and CCNE1 in one case each ( Fig. 1a ). No sequence alterations were found in the known melanoma oncogenes BRAF , NRAS , KIT , GNAQ or GNA11 or in any other of the 182 analyzed cancer-related genes. Figure 1: Genomic aberrations identified in 38 spitzoid neoplasms by targeted sequencing. ( a ) The columns denote the samples, the rows denote genes, brown squares represent gene fusions, red squares symbolize point mutations and indels, green squares denote gene amplifications and purple squares indicate truncating mutations. The identified fusion genes and HRAS mutations were mutually exclusive in 38 spitzoid neoplasms. Mutations in PKHD1, ERBB4 , LRP1B , and amplifications of MCL1 and CCNE1 are of unknown significance and co-occurred with kinase fusions and HRAS mutations. ( b ) Illustration of the distinct fusion genes for the ROS1 , ALK , NTRK1 , RET and BRAF rearrangements. The grey bars represent the exons of the genes, the numbers below the bars the exon number and the blue line the predicted breakpoints. The green shaded areas indicate the kinase domain and the blue shaded areas the coiled-coil domain of the fusion gene product. In the TP53–NTRK1 fusion transcript, multiple breakpoints spanning exon 8–12 of TP53 were predicted. Full size image Kinase fusions were identified in 18 of 30 (60%) Spitz naevi and in 6 of 8 (75%) atypical Spitz tumours ( Fig. 1a,b ). The rearrangements included gene fusions of the membrane-bound receptor tyrosine kinases ROS1 ( n =11, 29%), ALK ( n =6, 16%), NTRK1 ( n =3, 8%) and RET ( n =2, 5%). Two spitzoid neoplasms harboured t(7;19)(q34;q13) translocations that involved the serine/threonine kinase BRAF , but with different 5′-partners ( CEP89 and LSM14A ) in each tumour. Using reverse transcription polymerase chain reaction (RT–PCR) with breakpoint flanking primers, we verified that the fusion genes were expressed and produced in-frame transcripts. Using interphase fluorescence in situ hybridization (FISH) with breakpoint-flanking probes, we confirmed the disruptions at the ROS1 , ALK , NTRK1 , RET and BRAF loci. 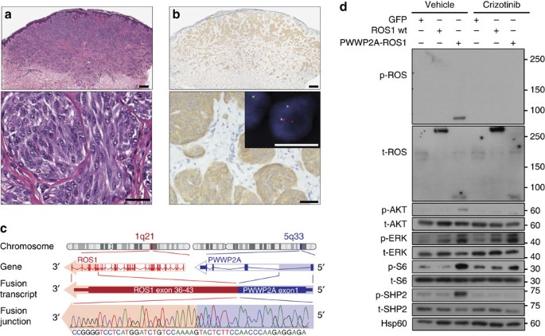Figure 2:ROS1fusions. (a) Histological section of an atypical Spitz tumour with aPWWP2A–ROS1fusion from the gluteal region of a 55-year-old female (haematoxylin and eosin stain). Scale bar, 500 μm. Scale bar magnification, 50 μm. (b) Immunohistochemistry for ROS1 shows expression in the melanocytes; stromal cells serve as internal negative controls. Scale bar, 500 μm. Scale bar magnification, 50 μm. The FISH inset confirms the gene rearrangements using breakpoint flanking FISH probes. The rearrangedROS1locus appears as individual green and red signals, and the wild-type kinase allele with juxtaposed green/red signals. Scale bar, 10 μm. (c) Illustration of thePWWP2A–ROS1kinase fusion.ROS1is located on chromosome 1q21, andPWWP2Aon chromosome 5q33. Owing to genomic rearrangements, exon 1 ofPWWP2Ais fused with exon 36–43 ofROS1, which contains the tyrosine kinase domain. The in-frame fusion junction of the transcript was confirmed by Sanger sequencing. (d) ThePWWP2A–ROS1fusion, but not the control-GFP construct, induces p-AKT, p-ERK, p-S6 and p-SHP2 in melan-a cells. Crizotinib inhibited at least partially the phosphorylation of the chimeric PWWP2A–ROS1 fusion protein, p-AKT, p-S6 and p-SHP2. The indicated protein weight markers in kDa are estimated from molecular weight standards. Results are representative of three independent experiments. We validated our findings in an independent cohort of 102 spitzoid neoplasms using interphase FISH ( Supplementary Table 2 summarizes the clinical, histopathological and genetic data). In total, we analysed 140 spitzoid neoplasms and identified fusions in 41 of 75 (55%) Spitz naevi, in 18 of 32 (56%) atypical Spitz tumours and in 13 of 33 (39%) spitzoid melanomas ( Table 1 ). We confirmed the expression of the chimeric ROS1, NTRK1, ALK and RET proteins using immunohistochemistry. Cases harbouring translocations showed moderate to strong staining for the corresponding fusion kinase, which was not observed in the cases lacking gene rearrangements. Patients with translocation-positive spitzoid neoplasms were younger (median 21 years) than patients whose tumours did not harbour translocations (median 32.5 years; Mann–Whitney test P <0.001). Table 1 Frequency of kinase fusions in spitzoid neoplasms. Full size table ROS1 fusions ROS1 rearrangements were found in 19 of 75 (25.3) Spitz naevi, 2 of 32 (6.3%) atypical Spitz tumours and 3 of 33 (9%) spitzoid melanomas ( Fig. 2a ). The ROS1 rearrangements fused the intact tyrosine kinase coding sequence of ROS1 to the 5′ portion of nine different partners ( Fig. 1b and Supplementary Figs 1–9 ). The expression of the chimeric ROS1 protein using immunohistochemistry was observed exclusively in cases with ROS1 rearrangements ( Fig. 2b,c ). Expression of the PWWP2A – ROS1 fusion construct in melan-a cells showed increased phosphorylation of the fusion protein, suggesting that the chimeric protein is constitutively active. Consistent with this, the MAPK and PI3K pathways were strongly activated compared with the green-fluorescent protein (GFP) and the wild-type, full-length ROS1 controls. The phosphorylation of PWWP2A–ROS1, AKT, S6 and SHP2, but not ERK, was at least partially inhibited by crizotinib, an Food and Drug Administration (FDA)-approved drug for lung cancer with ALK translocations that acts as an ALK [9] and ROS1 (ref. 12 ) inhibitor ( Fig. 2d ). Figure 2: ROS1 fusions. ( a ) Histological section of an atypical Spitz tumour with a PWWP2A – ROS1 fusion from the gluteal region of a 55-year-old female (haematoxylin and eosin stain). Scale bar, 500 μm. Scale bar magnification, 50 μm. ( b ) Immunohistochemistry for ROS1 shows expression in the melanocytes; stromal cells serve as internal negative controls. Scale bar, 500 μm. Scale bar magnification, 50 μm. The FISH inset confirms the gene rearrangements using breakpoint flanking FISH probes. The rearranged ROS1 locus appears as individual green and red signals, and the wild-type kinase allele with juxtaposed green/red signals. Scale bar, 10 μm. ( c ) Illustration of the PWWP2A – ROS1 kinase fusion. ROS1 is located on chromosome 1q21, and PWWP2A on chromosome 5q33. Owing to genomic rearrangements, exon 1 of PWWP2A is fused with exon 36–43 of ROS1 , which contains the tyrosine kinase domain. The in-frame fusion junction of the transcript was confirmed by Sanger sequencing. ( d ) The PWWP2A–ROS1 fusion, but not the control-GFP construct, induces p-AKT, p-ERK, p-S6 and p-SHP2 in melan-a cells. Crizotinib inhibited at least partially the phosphorylation of the chimeric PWWP2A–ROS1 fusion protein, p-AKT, p-S6 and p-SHP2. The indicated protein weight markers in kDa are estimated from molecular weight standards. Results are representative of three independent experiments. Full size image ALK fusions We found ALK fusions in 8 of 75 (10.7%) Spitz naevi, 5 of 32 (15.6%) atypical Spitz tumours and 1 of 33 (3%) spitzoid melanomas ( Fig. 3a ). Expression of the chimeric ALK protein was confirmed using immunohistochemistry and the rearrangements were validated in all cases with FISH ( Fig. 3b,c ). Cases without ALK rearrangements by sequencing did not show ALK expression by immunohistochemistry or separated signals by FISH. TPM3 and DCTN1 were 5′ fusion partners for ALK rearrangements ( Fig. 1b and Supplementary Figs 10 and 11 ). TPM3-ALK fusions were detected in eight spitzoid neoplasms. DCTN1 represents a novel fusion partner of ALK , was found in six cases, and resulted from a balanced translocation between homologous copies of chromosome 2 ( Fig. 3d ). Expression of the DCTN1–ALK fusion construct in melan-a cells showed increased phosphorylation of the fusion protein compared with the wild-type, full-length ALK , suggesting that the chimeric protein is constitutively active. Similar to the ROS1 fusions, AKT, ERK and S6 were more phosphorylated in melan-a cells with the ALK fusion construct compared with the GFP control. Crizotinib inhibited the ALK fusion-induced activation of the oncogenic PI3K and MAPK signalling pathways ( Fig. 3e ). 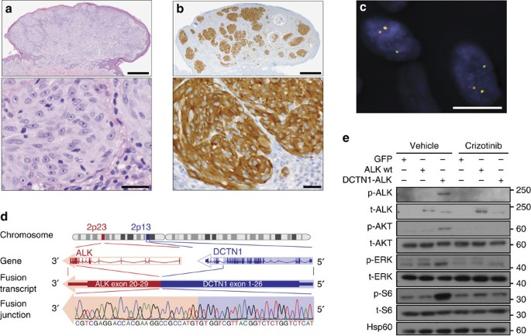Figure 3:ALKfusions. (a) Histological section of an atypical Spitz tumour with aDCTN1–ALKfusion excised from the upper arm of a 19-year-old male (haematoxylin and eosin stain). Scale bar, 500 μm. Scale bar magnification, 50 μm. (b) Immunohistochemistry shows ALK expression in the melanocytes; stromal cells serve as internal negative controls. Scale bar, 500 μm. Scale bar magnification, 50 μm. (c) FISH demonstrates theALKgene rearrangement by the individual green and orange signals using breakpoint flanking probes. Scale bar, 10 μm. (d) Illustration of theDCTN1–ALKkinase fusion.ALKis located on chromosome 2p23 andDCTN1on chromosome 2p13. Owing to genomic rearrangements, exon 1–26 ofDCTN1is fused with exon 20–29 ofALK, which contains the tyrosine kinase domain. The in-frame junction of the fusion transcript was confirmed with Sanger sequencing. (e) TheDCTN1–ALKfusion construct, but not the control-GFP construct, induces p-AKT, p-ERK and p-S6 in melan-a cells. These effects and the phosphorylation of chimeric DCTN1–ALK protein can be inhibited with crizotinib. The indicated protein weight markers in kDa are estimated from molecular weight standards. Results are representative of three independent experiments. Figure 3: ALK fusions. ( a ) Histological section of an atypical Spitz tumour with a DCTN1–ALK fusion excised from the upper arm of a 19-year-old male (haematoxylin and eosin stain). Scale bar, 500 μm. Scale bar magnification, 50 μm. ( b ) Immunohistochemistry shows ALK expression in the melanocytes; stromal cells serve as internal negative controls. Scale bar, 500 μm. Scale bar magnification, 50 μm. ( c ) FISH demonstrates the ALK gene rearrangement by the individual green and orange signals using breakpoint flanking probes. Scale bar, 10 μm. ( d ) Illustration of the DCTN1 – ALK kinase fusion. ALK is located on chromosome 2p23 and DCTN1 on chromosome 2p13. Owing to genomic rearrangements, exon 1–26 of DCTN1 is fused with exon 20–29 of ALK , which contains the tyrosine kinase domain. The in-frame junction of the fusion transcript was confirmed with Sanger sequencing. ( e ) The DCTN1–ALK fusion construct, but not the control-GFP construct, induces p-AKT, p-ERK and p-S6 in melan-a cells. These effects and the phosphorylation of chimeric DCTN1–ALK protein can be inhibited with crizotinib. The indicated protein weight markers in kDa are estimated from molecular weight standards. Results are representative of three independent experiments. Full size image NTRK1 fusions NTRK1 rearrangements were detected in 8 of 75 (10.7%) Spitz naevi, 8 of 32 (25%) atypical Spitz tumours and 7 of 33 (21.2%) spitzoid melanomas ( Fig. 4a ). The expression of NTRK1 was confirmed with immunohistochemistry in all cases with NTRK1 fusions ( Fig. 4b ), but was absent in cases without NTRK1 rearrangements. The LMNA–NTRK1 fusions involved the novel fusion partner LMNA (localized at 1q22) and were caused by a 743-kb deletion on chromosome 1q, joining the first two exons of LMNA with NTRK1 starting at exon 11 ( Fig. 4c ). The interchromosomal TP53–NTRK1 translocation resulted from a fusion joining NTRK1 starting from exon 9, containing the tyrosine kinase domain, to the 3′-untranslated region of TP53 ( Fig. 1b and Supplementary Figs 12,13 ). The expression of the LMNA–NTRK1 fusion construct in melan-a cells showed increased levels of phosphorylation of the fusion protein, AKT, ERK, S6 and PLCγ1 compared with the control cells. The strong activation of MAPK, PLCγ1 and PI3K pathways was inhibited by the NTRK1 inhibitor AZ-23 ( Fig. 4d ). 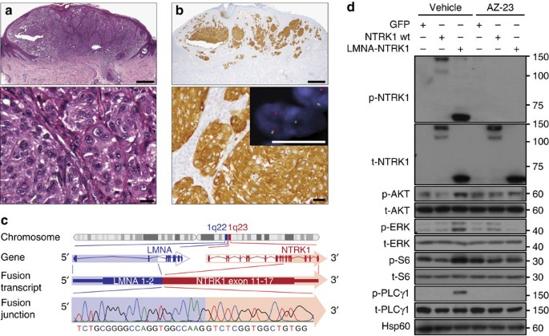Figure 4:NTRK1fusions. (a) Histological section of a spitzoid melanoma with aLMNA–NTRK1fusion excised from the left knee of a 39-year-old woman (haematoxylin and eosin stain). Scale bar, 500 μm. Scale bar magnification, 50 μm. (b) Immunohistochemistry demonstrates the NTRK1 expression in melanocytes; stromal cells serve as internal negative controls. Scale bar, 500 μm. Scale bar magnification, 50 μm. The FISH inset confirms the gene rearrangements using breakpoint flanking FISH probes by the individual green and red signals. Scale bar, 10 μm. (c) TheLMNA–NTRK1kinase fusion is caused by a 743 kb deletion on chromosome 1q, joining the first two exons ofLMNAwith exon 11–17 ofNTRK1.The in-frame junction of the fusion transcript was confirmed with Sanger sequencing. (d) TheLMNA–NTRK1fusion construct, but not the full-length, wild-type NTRK1 or the control-GFP constructs induce p-AKT, p-ERK, p-S6 and p-PLCγ1 in melan-a cells. A small molecule kinase inhibitor, AZ-23, inhibited the phosphorylation of LMNA–NTRK1 and the activation of the oncogenic signalling pathways. The indicated protein weight markers in kDa are estimated from molecular weight standards. Results are representative of three independent experiments. Figure 4: NTRK1 fusions. ( a ) Histological section of a spitzoid melanoma with a LMNA–NTRK1 fusion excised from the left knee of a 39-year-old woman (haematoxylin and eosin stain). Scale bar, 500 μm. Scale bar magnification, 50 μm. ( b ) Immunohistochemistry demonstrates the NTRK1 expression in melanocytes; stromal cells serve as internal negative controls. Scale bar, 500 μm. Scale bar magnification, 50 μm. The FISH inset confirms the gene rearrangements using breakpoint flanking FISH probes by the individual green and red signals. Scale bar, 10 μm. ( c ) The LMNA – NTRK1 kinase fusion is caused by a 743 kb deletion on chromosome 1q, joining the first two exons of LMNA with exon 11–17 of NTRK1. The in-frame junction of the fusion transcript was confirmed with Sanger sequencing. ( d ) The LMNA–NTRK1 fusion construct, but not the full-length, wild-type NTRK1 or the control-GFP constructs induce p-AKT, p-ERK, p-S6 and p-PLCγ1 in melan-a cells. A small molecule kinase inhibitor, AZ-23, inhibited the phosphorylation of LMNA–NTRK1 and the activation of the oncogenic signalling pathways. The indicated protein weight markers in kDa are estimated from molecular weight standards. Results are representative of three independent experiments. Full size image RET fusions We found RET fusions in 2 of 75 (2.7%) Spitz naevi, 1 of 32 (3.1%) atypical Spitz tumours and 1 of 33 (3%) spitzoid melanomas ( Fig. 5a ). Fusions of RET on chromosome 10q11 involved the 5′ fusion partners KIF5B on chromosome 10p11 and GOLGA5 on chromosome 14q32 ( Fig. 1b and Supplementary Figs 14,15 ). In both fusions, the RET tyrosine kinase domain was fused to the coiled-coil domains of KIF5B (exons 1–16) or GOLGA5 (exons 1–7). Immunohistochemical expression of RET was observed only in cases with RET translocations ( Fig. 5b ). Expression of the GOLGA5–RET fusion construct in melan-a cells showed increased phosphorylation of the fusion protein, AKT, ERK, S6 and PLCγ-1 compared with control cells. The phosphorylation of these proteins could be suppressed by vandetanib ( Fig. 5c ) or cabozantinib ( Fig. 5d ), which are both small molecule RET inhibitors that are FDA-approved for medullary thyroid cancer. 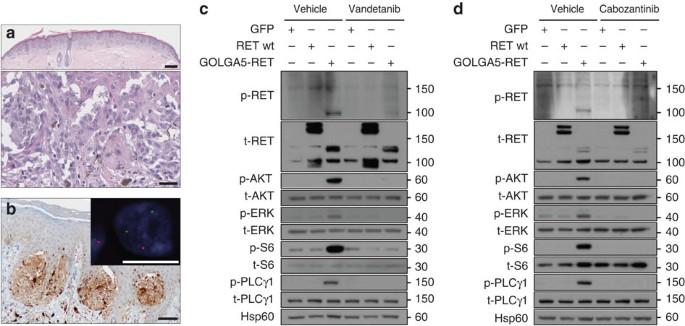Figure 5: RET fusions. (a) Histological section of a pigmented spindle cell naevus (a morphological variant of Spitz naevus) with aGOLGA5–RETfusion excised from a 50-year-old woman (haematoxylin and eosin stain). Scale bar, 500 μm. Scale bar magnification, 50 μm. (b) RET expression in melanocytes; keratinocytes serve as internal negative controls. Scale bar, 100 μm. The individual green and red signals in FISH confirm the gene rearrangements using breakpoint flanking FISH probes. Scale bar, 10 μm. (c,d) TheGOLGA5–RETconstruct, but not the wild-type, full-length RET or the control-GFP constructs induces p-AKT, p-ERK, p-S6 and p-PLCγ1 in melan-a cells. The activation of these pathways and the phosphorylation of GOLGA5–RET can be inhibited with (c) vandetanib and (d) cabozantinib. The indicated protein weight markers in kDa are estimated from molecular weight standards. Results are representative of three independent experiments. Figure 5: RET fusions. ( a ) Histological section of a pigmented spindle cell naevus (a morphological variant of Spitz naevus) with a GOLGA5–RET fusion excised from a 50-year-old woman (haematoxylin and eosin stain). Scale bar, 500 μm. Scale bar magnification, 50 μm. ( b ) RET expression in melanocytes; keratinocytes serve as internal negative controls. Scale bar, 100 μm. The individual green and red signals in FISH confirm the gene rearrangements using breakpoint flanking FISH probes. Scale bar, 10 μm. ( c , d ) The GOLGA5–RET construct, but not the wild-type, full-length RET or the control-GFP constructs induces p-AKT, p-ERK, p-S6 and p-PLCγ1 in melan-a cells. The activation of these pathways and the phosphorylation of GOLGA5–RET can be inhibited with ( c ) vandetanib and ( d ) cabozantinib. The indicated protein weight markers in kDa are estimated from molecular weight standards. Results are representative of three independent experiments. Full size image BRAF fusions We identified gene rearrangements of the serine/threonine kinase BRAF in 4 of 75 (5.3%) Spitz naevi, 2 of 32 (6.3%) atypical Spitz tumours and 1 of 33 (3%) spitzoid melanomas. The fusion genes contained CEP89 exons 1–16 followed by the kinase domain of BRAF encoded by exons 9–18, or LSM14A exons 1–9 followed by BRAF exons 9–18, both resulting in loss of the auto-inhibitory, N-terminal RAS-binding domain of BRAF ( Fig. 1b and Supplementary Figs 16,17 ). In addition to the identified translocations, 1 of 75 (1.3%) Spitz naevi and 1 of 32 (3.1%) atypical Spitz tumours showed BRAF amplification as determined by at least eight BRAF fusion signals per nucleus in interphase FISH. Functional validation in xenograft models To validate the oncogenic roles of the novel fusion kinases, we stably transduced mouse melan-a cells with PWWP2A–ROS1, DCTN1–ALK, LMNA–NTRK1 , and GOLGA5–RET fusions. We then injected the transduced cells subcutaneously and bilaterally into the flanks of immunocompromised mice. We monitored the mice for tumour formation every 3–4 days. Within 40 days, all injection sites in the fusion kinase groups ( PWWP2A–ROS1, DCTN1–ALK, LMNA–NTRK1, GOLGA5–RET ) developed rapidly growing tumours similarly to those observed at the injection sites of melanocytes expressing the known melanoma oncogenes HRAS G12V and NRAS G12V ( Supplementary Fig. 18 ). We observed no tumours at the injection sites in the control group with melanocytes that had been transduced with GFP. Our results show that kinase fusions are important mechanisms of oncogene activation in spitzoid neoplasms. In aggregate, 72 of 140 (51%) spitzoid neoplasms harboured fusions involving the receptor tyrosine kinases ROS1 (17%), NTRK1 (16%), ALK (10%), RET (3%) and the serine/threonine kinase BRAF (5%). All fusions occurred in a mutually exclusive pattern ( Fig. 1a ), and no fusions were detected in tumours with HRAS mutations. All of the sequenced kinase fusions created chimeric proteins that retained the intact kinase domain at the 3′ end of the fusion transcript ( Fig. 1b ), a pattern similar to that observed in other cancers that harbour rearrangements involving these kinases [13] , [14] , [15] . All recombination sites between kinases and translocation partners involved the canonical intronic recombination sites, similar to those described in other types of cancers ( ROS1 : introns 33–35; ALK : intron 19; NTRK1 : introns 8–10; RET : intron 11; BRAF : intron 8) [16] . The majority of the novel 5′ fusion partners identified in our study, namely those of ROS1 ( PWWP2A , PPFIBP1 , ERC1 , MYO5A , CLIP1 , HLA-A , KIAA1598 and ZCCHC8 ), ALK ( DCTN1 ), NTRK1 ( LMNA ) and BRAF ( CEP89 and LSM14A ) contributed coiled-coil domains to the fusion proteins. The coiled-coil domains may play similar roles to the established 5′ fusion partners ( TPM3 (ref. 17 ), GOLGA5 (ref. 18 ), KIF1B [13] ) of these kinases in promoting dimerization [19] and auto-activation of the kinases [20] . Rearrangements of the kinases ROS1 , ALK , NTRK1 , RET and BRAF with similar fusion sites have previously been described in various types of aggressive tumours. ROS1 fusions have been described in various cancer types, including lung carcinoma [21] , glioblastoma [22] and cholangiocarcinoma [23] . ALK fusions have been described in anaplastic large cell lymphoma [17] , lung cancer [14] , inflammatory myofibroblastic tumour [24] and anecdotal studies have also reported ALK fusions in acral melanoma [25] . RET fusions, including the pericentric inversions giving rise to the KIF5B–RET fusion observed in spitzoid neoplasms, have been shown to drive lung cancer formation [13] , [15] , [26] and an interchromosomal GOLGA5–RET rearrangement was first described in papillary thyroid carcinomas occuring in children exposed to radioactive fallout from the Chernobyl nuclear accident [18] . BRAF fusions have been identified in pilocytic astrocytomas [27] , papillary thyroid carcinoma [28] and rarely in melanocytic tumours [29] , [30] . In addition, our data shows that patients with translocation-positive spitzoid neoplasms were younger than patients whose tumours lacked translocations are similar to observations that lung cancers [15] , thyroid cancers [18] and astrocytomas [27] harbouring kinase fusions are more common in younger patients. Our findings of the activated effector pathways downstream of the fusion kinases are in line with other experimental systems of cancer. For example, ubiquitous expression of constitutively active RFP–RET fusions in mice results in generalized melanocyte proliferation, formation of naevi and ultimately melanomas with MAPK pathway activation; this is similar to our finding of GOLGA5–RET fusions in spitzoid neoplasms [31] . Autocrine neurotrophin signalling involving NTRK1 has been shown to promote proliferation and migration in melanoma cell lines [32] , and constitutively active NTRK1 activates the MAPK and PI3K pathways in NIH-3T3 cells [33] . Phosphorylation of the MAPK and PI3K pathways is an essential component of oncogenic ALK signalling in lymphoma [17] and lung cancer [14] , and we found that the novel fusion DCTN1–ALK has similar effects. The activation of the MAPK and PI3K pathways by the novel PWWP2A–ROS1 fusion is also similar to the changes associated with other oncogenic ROS1 fusions in various cancer types [12] , [34] . The results of our functional validation experiments in xenograft models are consistent with previous studies, which showed that TPM3-ROS1 (ref. 15 ) , EML4-ALK [14] and KIF5B - RET [13] , [15] , [26] fusions drive tumour formation in non-small cell lung cancers. The common occurrence of kinase fusions in the entire biologic spectrum of spitzoid neoplasms (benign Spitz naevi, atypical Spitz tumours and spitzoid melanomas) suggests that these fusions occur early in the pathogenesis of spitzoid neoplasms. Therefore, kinase fusions are necessary but not sufficient for malignant transformation—a situation analogous to that of mutations in oncogenes (such as BRAF , NRAS , GNAQ and GNA11 ) commonly found in melanocytic neoplasms. Consequently, the frequent kinase fusions described herein are unlikely to be useful in distinguishing benign from malignant spitzoid neoplasms. Although the majority of spitzoid neoplasms behave in an indolent manner, some spitzoid tumours metastasize and require systemic therapy. Lung cancers, lymphomas and sarcomas with ALK or ROS1 fusions, and thyroid cancers with RET fusions can be successfully treated using US FDA-approved kinase inhibitors such as crizotinib, cabozantinib and vandetanib. The fusion kinases identified here are therefore potential therapeutic targets for translocation-positive melanocytic tumours that require systemic therapy. Patients The study was conducted according to the Declaration of Helsinki, and human tissues were obtained with patient-informed consent under approval by the Institutional Review Boards/Ethics Committees of Memorial Sloan-Kettering Cancer Center, New York, the University of California, San Francisco, and the Medical University of Graz, Austria. The excised skin lesions were fixed in 4% neutral-buffered formalin, embedded in paraffin, processed using routine histological methods and stained with haematoxylin–eosin. Specimens were collected over a time period of 6 months and the histopathologic diagnosis of Spitz naevus, atypical Spitz tumour and spitzoid melanoma was confirmed by at least three dermatopathologists. Specimens with insufficient tissue amount or severely degraded nucleic acids were excluded. In total, specimens from 140 patients were analysed and the clinical, histologic and genetic characteristics are summarized in Supplementary Tables 1,2 . Targeted DNA sequencing We sequenced 3,230 exons from 182 cancer-related genes ( Supplementary Table 3 ) and 37 introns of 14 ( Supplementary Table 4 ) commonly rearranged genes in cancer with average depth-of-coverage of greater than 500 × . Prior to DNA extraction, FFPE samples from all cases were reviewed to confirm that the tissue was of sufficient size to generate a minimum of 50 ng of DNA and that this DNA would be derived from areas that contained a minimum of 20% melanocytic nuclei. DNA was isolated from 40-μm-thick sections of FFPE tissue. DNA sequencing was performed on indexed, adaptor ligation, hybridization-captured libraries (Agilent SureSelect custom kit). Sequencing was performed on the HiSeq-2000 instrument (Illumina), with 49 × 49 paired reads to an average depth of 997 × ( Supplementary Table 5 ). RNA sequencing Total RNA extracted from the 40-μm-thick sections of FFPE tumour was reverse-transcribed with random hexamer primers using the SuperScript III First-Strand Synthesis System (Invitrogen). Double-stranded cDNA was synthesized with the NEBNext mRNA Second Strand Synthesis Module (New England Biolabs) [35] . Hybrid selection of indexed, adaptor-ligated libraries was performed using the cDNA Kinome hybridization kit with 612 transcripts of kinases and kinase-related genes (Agilent SureSelect Human Kinome Kit). [36] Selected libraries were sequenced on the HiSeq-2000 instrument (Illumina) with 49 × 49 paired reads. For RNA sequencing, we used a sequencing approach targeting 612 transcripts of kinases and kinase-related genes. We aimed for a high number of unique read pairs (≥50,000,000) per sample ( Supplementary Table 6 ). Sequence data analysis Sequence data from gDNA and cDNA were mapped to the reference human genome (hg19) using the BWA aligner and processed using publically available SAMtools [37] , Picard ( http://picard.sourceforge.net ) and GATK [38] . Genomic base substitutions and indels were detected using custom tools optimized for mutation calling in heterogeneous tumour samples, based on detecting common sequence variations and local sequence assembly. Variations were filtered using Single Nucleotide Polymorphism Database and a custom artifact database, and then annotated for known and likely somatic mutations using COSMIC. Copy number alterations were detected by comparing targeted genomic DNA sequence coverage with a process-matched normal control sample. Genomic rearrangements were detected by clustering chimeric reads mapping to targeted introns/exons. Expression levels were determined by analysing cDNA sequence coverage of targeted exons. Gene fusion confirmation All gene fusions were validated with qRT–PCR from cDNA using the primers listed in Supplementary Table 7 and analysis on a Bioanalyzer (Agilent). Specific PCR amplicons were only detected with the appropriate combination of primers and template, and not with negative controls. The nucleotide sequence at the fusion site was confirmed with Sanger sequencing. Interphase fluorescence in situ hybridization A commercially available break-apart probe was used for ALK according to the manufacturer’s protocol (Abbott, Des Plaines, IL). For ROS1 , RET , NTRK1 and BRAF , break-apart FISH probes were prepared from BAC clones using standard procedures and labelled by nick translation with SpectrumGreen-dUTP and SpectrumRed-dUTP (Abbott). The following flanking BAC clones were used: RET (red: RP11-379D20, RP11-124O11; green: RP11-718J13, RP11-54P13), NTRK1 (red: RP11-284F21, RP11-66D17; green: RP11-1038N13, RP11-1059C21), ROS1 (red: RP11-379F24, RP11-103F10; green: RP11-1059G13, RP11-721K11) and BRAF (red: RP11-715H9, RP11-133N19; green: RP11-759K14, RP11-788O6). The probes were hybridized on 5-μm-thick tissue sections, and the number and localization of the hybridization signals were assessed in a minimum of 100 interphase nuclei with well-delineated contours and at least 50% of neoplastic cells had to show a split signal to report a rearrangement of a kinase. Immunohistochemistry Immunohistochemical analysis was performed on archival FFPE tumour specimens to confirm the expression of the fusion kinases and the activation of oncogenic pathways. We used a Discovery Ultra instrument with a multimer/DAB detection system (Ventana Medical Systems Inc., Tucson, AZ, USA) with appropriate negative and positive controls the following antibodies: ALK (clone D5F3; Cell Signalling, Danvers, MA, USA; dilution: 1:250), ROS1 (clone D4D6; Cell Signalling; dilution: 1:25), NTRK1 (clone EP1058Y; Epitomics, Burlingame, CA, USA; dilution: 1:100), RET (clone EPR287; Epitomics; dilution: 1:250). The percentage of tumour cells exhibiting staining was scored by at least two independent pathologists. Plasmids To investigate the functional roles and the activation of oncogenic signalling pathways, we cloned PWWP2A–ROS1, DCTN1–ALK, LMNA–NTRK1 and GOLGA5–RET fusions and expressed them in melan-a cells (immortalized, non-tumourigenic mouse melanocytes). Expression vectors with GFP and the full-length, wild-type kinases ROS1 , ALK , NTRK1 and RET were used as controls. Plasmids containing cDNAs of the genes of interest were obtained ( Supplementary Table 8 ) and their sequences were verified [39] , [40] , [41] . Non-synonymous mutations deviating from the RefSeq sequence found in the NTRK1 and RET plasmids were corrected using QuikChange site-directed mutagenesis (Agilent Technologies). Fusion constructs were generated by overlap extension [42] . Once PCR products containing the target cDNAs were generated, they were cloned into a pENTR vector using the pENTR/D-TOPO cloning kit (Life Technologies). All constructs were subsequently cloned into the pLenti6.3/TO/V5-Dest backbone (Life Technologies) and checked by digestion and sequencing. The larger fusion genes involving ALK and ROS1 were also cloned into the PBX2.1 backbone of the PiggyBac Transposon system [43] . Stably transduced melan-a cells Melan-a cells were generously provided by Dr Dorothy C Bennett (St George’s Hospital, University of London, London, UK) [44] and maintained in glutamine-containing RPMI-1640 supplemented with 10% heat-inactivated foetal bovine serum, 200 nM of 12-O-tetradecanoylphorbol-13-acetate, penicillin (100 units ml −1 ) and streptomycin (50 mg ml −1 ). 293FT cells were purchased from Life Technologies and maintained in DME-H21 medium containing 10% heat-inactivated foetal bovine serum, MEM Non-Essential Amino Acids (0.1 mM), sodium pyruvate (1 mM), penicillin (100 units ml −1 ) and streptomycin (50 mg ml −1 ). Lentiviruses were produced by transfecting 293FT cells with plasmid DNA in a pLenti6.3/TO/V5-Dest backbone together with ViraPowerTM (Life Technologies) according to the manufacturer’s protocol. Infections of melan-a cells were conducted in the presence of 10 μg ml −1 of Polybrene (Santa Cruz Biotechnology, Santa Cruz, CA, USA). Stably transduced melan-a cells expressing GOLGA5–RET , LMNA–NTRK1 , PWWP2A–ROS1 , RET and NTRK1 were generated by infection with the respective lentivirus. ALK and ROS1 expressing melan-a cell lines were generated by cotransfection of the PBX2.1 construct together with pCMV-HyPBase transposase vector. Melan-a cell lines stably expressing GFP were generated using pLenti6.2/V5 and PBX2.1 vectors and were used as a control. Cells were selected for at least 20 days using 5 μg ml −1 of blasticidin S-hydrochloride (Life Technologies) after transduction. Western blotting Anti-RET (no. 3220), anti-phospho-RET (Tyr905) (no. 3221), anti-ALK (no. 3791), anti-phospho-ALK (Tyr1096) (no. 6962), anti-ROS1 (no. 3266), anti-phospho ROS1 (Tyr2274) (no. 3078), anti-phospho-p44/42 MAPK (Erk1/2) (Thr202/Tyr204) (no. 9101), anti-AKT (no. 9272), anti-phospho-AKT (Ser473) (no. 9271), anti-S6 Ribosomal Protein (no. 2317), anti-phospho-S6 Ribosomal Protein (Ser235/236) (no. 2211), anti-PLCγ1 (no. 2822), anti-phospho-PLCγ1 (Tyr783) (no. 2821), anti-SHP2 (D50F2) (no. 3397), anti-phospho-SHP2 (Tyr 542) (no. 3751), as well as the secondary antibodies anti-rabbit IgG-HRP (no. 7076) and anti-mouse IgG-HRP (no. 7074) were purchased from Cell Signalling Technology. Anti-HSP60 (sc-1722) and anti-ERK2 (C-14) (sc-154) as well as the secondary antibodies anti-goat IgG-HRP (sc-2033) were purchased from Santa Cruz Biotechnology. Anti-TrkA (ab37837) and anti-phospho-TrkA (Tyr408) (ab1445) were purchased from Abcam (Cambridge, MA, USA). Cell lysates were prepared in RIPA buffer supplemented with Halt protease and phosphatase inhibitor cocktail (Thermo Scientific). Equal amounts of protein, as measured by BCA protein assay, were resolved in 4–12% Bis-Tris NuPage gradient gels (Life Technologies) and transferred electrophoretically on a polyvinylidene difluoride 0.45-μ membrane. Membranes were blocked for 1 h at room temperature in 5% bovine serum albumin (BSA) or non-fat milk in TBST before being incubated overnight at 4 °C with the primary antibodies. All primary antibodies were diluted 1:1,000 in 5% BSA or non-fat milk in TBST. After three washes of 5 min in TBST, secondary antibodies were diluted 1:3,000 in 5% non-fat milk in TBST and incubated for 1 h at room temperature. After another three washes in TBST, detection of the signal was achieved by incubating the membrane on an ECL solution from Millipore and exposure on autoradiography films from Denville Scientific (Metuchen, NJ, USA). The full blots are shown in Supplementary Figs 19–23 . Drug studies Vandetanib and cabozantinib were purchased from Selleckchem (Houston, TX, USA). Crizotinib was purchased from Chemie Tek (Indianapolis, IN, USA). AZ-23 was purchased from Axon Medchem (Groningen, The Netherlands). Tumourigenicity study Animal experiments were carried out in accordance with the Declaration of Helsinki and were approved by the ethical committee of the University of California, San Francisco. A total of 1.5 million melan‐a cells stably transduced with the indicated oncogene or GFP control vector were injected subcutaneously in two separate, 6-week-old female nonobese diabetic/severe combined immunodeficiency, interleukin 2-Rγ null mice. Mice were palpated three times a week for the development of tumours over a period of 40 days. How to cite this article: Wiesner, T. et al . Kinase fusions are frequent in Spitz tumours and spitzoid melanomas. Nat. Commun. 5:3116 doi: 10.1038/ncomms4116 (2014). Accession codes: Sequence data have been deposited in the GenBank sequence read archive (SRA) under the accession code SRP033273 .